Harvesting singlet fission for solar energy conversion via triplet energy transfer The efficiency of a conventional solar cell may be enhanced if one incorporates a molecular material capable of singlet fission, that is, the production of two triplet excitons from the absorption of a single photon. To implement this, we need to successfully harvest the two triplets from the singlet fission material. Here we show in the tetracene (Tc)/copper phthalocyanine (CuPc) model system that triplets produced from singlet fission in the former can transfer to the later on the timescale of 45±5 ps. However, the efficiency of triplet energy transfer is limited by a loss channel due to faster formation (400±100 fs) and recombination (2.6±0.5 ps) of charge transfer excitons at the interface. These findings suggest a design principle for efficient energy harvesting from singlet fission: one must reduce interfacial area between the two organic chromophores to minimize charge transfer/recombination while optimizing light absorption, singlet fission and triplet rather than singlet transfer. The efficiency of a conventional solar cell based on a single semiconductor material is constrained by the Shockley–Queisser limit (~31%) because the excess photon energy above the bandgap of the semiconductor is lost as heat [1] . Among the proposals to exceed this limit is to convert part of the excess photon energy to the excitation of multiple electron-hole pairs in a process called multiple exciton generation or singlet fission, with the new power conversion efficiency as high as 44% (ref. 2 ). Singlet fission is particularly attractive because of the high quantum efficiency (~200%, triplet excitons per photon) in a few well-known organic semiconductors, such as pentacene and Tc, and the prospect of designing and synthesizing new singlet fission molecules [3] , [4] . Although several research groups have demonstrated solar cells and photodetectors using singlet fission materials [5] , [6] , [7] , [8] , [9] , [10] , we are far from understanding how to efficiently harvest singlet fission for enhanced solar energy conversion. Design principles for molecules with high singlet fission yields are starting to emerge [3] , [4] but little is known about how to optimally extract the two electron-hole pairs resulting from singlet fission. This is a complex process involving the dynamic competition of singlet fission and two electron transfer (from the triplet pair) with channels such as radiative or non-radiative recombination, intersystem crossing, and energy transfer or charge transfer (CT) from the singlet. One strategy of harvesting singlet fission for solar energy conversion is to form an interface between a singlet fission material (for example, Tc or pentacene) and an electron acceptor (for example, fullerene or inorganic semiconductor quantum dots) for multiple CT (refs 5 , 6 , 7 , 8 , 9 , 10 ). A limitation of this approach is that CT processes from both the singlet and the triplet pair are possible [11] ; the former does not contribute to any increase in power conversion efficiency beyond the Shockley–Queisser limit and is difficult to avoid for most electron acceptors. Another difficulty is that the electron (or hole) acceptor material may not necessarily serve as an efficient light absorber in the long wavelength region, as required for a singlet fission solar cell. To circumvent the difficulties presented above, one may couple a singlet fission material (A) and a second chromophore (B) absorbing at longer wavelength with a common electron acceptor (C) [5] , [7] . Triplet excitons generated via singlet fission in A can transfer through B to reach the interface with C for charge collection. This approach takes advantage of the flexibility of the two chromophores (A and B) to better cover the solar spectrum. It avoids the direct interface between the singlet fission material and the electron acceptor, thus, in principle, eliminating the less efficient channel of electron transfer from singlet excitons in A to C (ref. 11 ). This scheme is enabled by the relatively long-lived triplet excitons [12] that can be transferred over long distances [13] from A through B before eventually reaching the charge-separating interface with C. Recently, Baldo and co-workers used the Tc/CuPc/C 60 trilayer structure and suggested the transport of triplets from singlet fission in Tc through the CuPc layer to reach C 60 for enhanced photocurrent, but the overall power conversion efficiency of the device remained low [7] . Here we show in the model system of Tc/CuPc bilayers that while triplet energy transfer does occur on timescales expected for triplet diffusion, having the donor/donor interface also introduces a competitive channel due to CT and recombination from singlet exciton dissociation at the interface. This channel is unfortunately a consequence of the energetic requirement necessary for efficient triplet energy transfer from the singlet fission material to the second chromophore. Minimizing this loss channel is thus critical to singlet fission solar cells based on triplet energy transfer and multiple charge collection. The model system and energetic alignment We choose the model system of Tc/CuPc because these two materials may satisfy the energetic requirement proposed for a trilayer singlet fission solar cell ( Fig. 1 ) where triplets produced by singlet fission in Tc (a) may in principle transfer through CuPc (b) to reach the interface with the electron acceptor C 60 (c). Singlet fission in crystalline Tc is known to be efficient with quantum yields (for triplets) as high as 200% (refs 3 , 4 ). The reported time scales for singlet fission in crystalline Tc vary broadly [3] , [4] , [14] , with recent studies converging to 50–80 ps (refs 15 , 16 ). We have examined singlet fission in Tc thin films using time-resolved two-photon photoemission (TR-2PPE) spectroscopy and discovered a quantum coherent mechanism in which optical excitation of the singlet results in a quantum superposition between the singlet state and the multiexciton state (ME) also called a correlated triplet pair [17] . The quantum superposition in Tc possesses a lifetime of 7 ps (refs 11 , 17 ) after which the triplet pair state decouples from the singlet. The triplet excitation energy in Tc is T 1 =1.25 eV (refs 15 , 16 , 17 ) and that in CuPc is T′ 1 =1.15 eV (ref. 18 ); the near-resonant but slightly downhill energetics should facilitate efficient triplet energy transfer from Tc to CuPc. The optical absorption spectrum of CuPc is ideally complementary to that of Tc, as shown in Fig. 2a . This allows us to selectively excite either Tc or CuPc in a bilayer film. 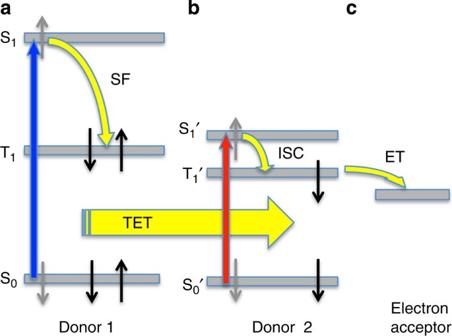Figure 1: Schematic of a trilayer strategy for the harvesting of singlet fission. (a) Singlet fission (SF) donor absorbing in the blue region, (b) donor 2 absorbing in the red, and (c) a common electron acceptor. The blue and red arrows represent photons with high and low energies, respectively. The yellow arrows represent SF, triplet energy transfer (TET), intersystem crossing (ISC) and electron transfer (ET). Figure 1: Schematic of a trilayer strategy for the harvesting of singlet fission. ( a ) Singlet fission (SF) donor absorbing in the blue region, ( b ) donor 2 absorbing in the red, and ( c ) a common electron acceptor. The blue and red arrows represent photons with high and low energies, respectively. The yellow arrows represent SF, triplet energy transfer (TET), intersystem crossing (ISC) and electron transfer (ET). 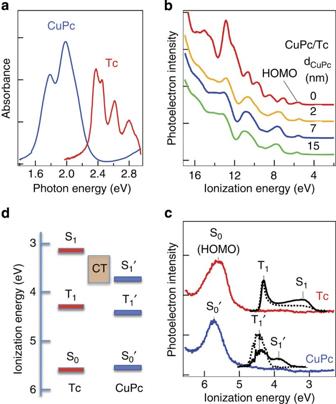Figure 2: Electronic energy alignment at the interface. (a) Optical absorption spectra of solid thin films (~20 nm) of tetracene (Tc, red) and copper phthalocyanine (CuPc, blue); (b) UPS of a 20-nm Tc thin film with CuPc overlayer thicknessdCuPc=0 (red), 2 (orange), 7 (blue) and 15 (green) nm. Thexaxis is ionization energy (Evac−E) and Evacis the vacuum level; (c) UPS for Tc (red, 20 nm) and CuPc (blue, 15 nm), along with TR-2PPE spectra integrated in two time windows (solid, −0.5 to 1 ps; dashed, 9–10 ps). (d) An energy level alignment diagram for the excitonic states in Tc (red) and CuPc (blue). The light brown region represents CT excitons across the CuPc/Tc interface. Full size image Figure 2: Electronic energy alignment at the interface. ( a ) Optical absorption spectra of solid thin films (~20 nm) of tetracene (Tc, red) and copper phthalocyanine (CuPc, blue); ( b ) UPS of a 20-nm Tc thin film with CuPc overlayer thickness d CuPc =0 (red), 2 (orange), 7 (blue) and 15 (green) nm. The x axis is ionization energy (E vac −E) and E vac is the vacuum level; ( c ) UPS for Tc (red, 20 nm) and CuPc (blue, 15 nm), along with TR-2PPE spectra integrated in two time windows (solid, −0.5 to 1 ps; dashed, 9–10 ps). ( d ) An energy level alignment diagram for the excitonic states in Tc (red) and CuPc (blue). The light brown region represents CT excitons across the CuPc/Tc interface. Full size image We first use one-photon ultraviolet photoemission spectroscopy (UPS) to determine the interfacial alignment of valence electronic structures. Figure 2b shows UPS of CuPc with different thickness (0–15 nm) deposited on top of a 20-nm Tc thin film. The position of the highest occupied molecular orbital (HOMO) is indicated. For neat Tc, the spectrum is characterized by the HOMO (5.6±0.1 eV), HOMO- n ( n =1, 2,…) and other deeper valence bands [19] . With the deposition of CuPc on top of the Tc thin film, the spectrum changes to that of CuPc (ref. 20 ); even for CuPc film thickness of 2 nm, spectral features associated with the underlying Tc layer are negligible, as expected from the small escape depth of photoelectrons. The ionization energy of the CuPc HOMO is 5.5±0.1 eV for the bilayer sample, indicating near-resonant condition for hole transfer at the CuPc/Tc interface. Here we use peak positions in UPS for easy comparison with photoelectron spectra of optically excited states from 2PPE, as sources of broadening may be very different in these two spectroscopy methods. Note that threshold energies in UPS are usually preferred when one compares transport levels [20] . Figure 2c shows TR-2PPE spectra for neat Tc and CuPc, along with the S 0 region of corresponding UPS. In a TR-2PPE experiment, the material is first excited by the pump photon (hν 1 =2.43 and 1.96 eV for Tc and CuPc, respectively) to create excitonic states. After a controlled time delay, the excitonic states are ionized and the photoelectrons detected. For each surface, we show two TR-2PPE spectra integrated for different time windows. At short times (−0.5 to −1 ps), the TR-2PPE spectrum for either Tc or CuPc shows the presence of both singlet (S 1 ) and triplet ( T 1 ) states. At longer times (9–10 ps), T 1 dominates each spectrum. The energy level alignment of all excitonic levels involved is summarized schematically in Fig. 2d . The ionization energies of CuPc S 0 is ~0.1 eV smaller than that of Tc. The ionization energies of T 1 and S 1 states in Tc are smaller than those in CuPc by 0.1 and 0.7 eV, respectively. Note that smaller ionization energy for an excitonic state means higher excitation energy (referenced to S 0 ). The use of ionization energy scale is particularly helpful when we consider electron transfer from excitonic states, as the ionization of any of these states leaves behind a common final state, a hole in the HOMO of the donor molecule. On the scale of ionization energy referenced to the vacuum level (E vac −E), the HOMO level is equivalent to the ionization energy of the ground S 0 state. Interfacial CT and recombination The large difference in S 1 energy between Tc and CuPc, along with the resonant nature of the HOMO levels, suggests that the lowest unoccupied molecular orbitals are similarly offset, provided that the exciton-binding energies in these two molecules are similar. Thus, electron transfer from the S 1 state of Tc to the lowest unoccupied molecular orbital level of CuPc, leading to the formation of a CT exciton, is energetically favourable. Indeed, the transient formation of interfacial CT excitons (tan region in the schematics, Fig. 2d ) is observed in TR-2PPE spectroscopy, as we detail below. Two bilayer samples are used: 2 nm CuPc on 2 nm Tc and 2 nm CuPc on 20 nm Tc. In the TR-2PPE experiment, the pump photon energy (hν 1 =2.43 eV) is chosen to selectively photoexcite Tc, not CuPc. After a controlled time delay, the probe photon (hν 2 =4.65 eV) ionizes each excitonic state for detection. The surface sensitivity of the photoemission technique, along with the thin CuPc overlayer used in the experiment, allows us to focus on interfacial charge and energy transfer dynamics with minimal complication from transport in the CuPc phase. 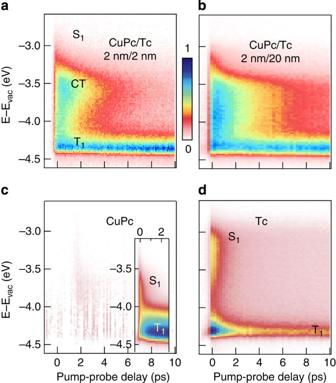Figure 3: Pseudo-colour plots of TR-2PPE spectra in 10 ps. (a) 2 nm CuPc on 2 nm tetracene (Tc); (b) 2 nm CuPc on 20 nm Tc; (c) 15 nm CuPc only; and (d) 20 nm of Tc only. The colour scale represents photoemission intensity (normalized). All spectra were recorded with hν1=2.43 eV and hν2=4.65 eV. The inset incshows TR-2PPE spectra for the 15-nm CuPc thin film excited at hν1=1.96 eV and probed at hν2=4.65 eV. Figure 3a,b presents pseudo-colour plots of TR-2PPE spectra for the bilayer samples. Here the photoelectron intensity is a sum of contributions from excitations within the Tc bottom layer and from charge/energy transfer to CuPc at the interface. The two spectra are similar. Each is dominated by the triplet (T 1 ) peak with nearly constant intensity on this timescale (0–10 ps) and a broad and transient peak around −3.6 eV (below E vac ), which we label as CT. Figure 3: Pseudo-colour plots of TR-2PPE spectra in 10 ps. ( a ) 2 nm CuPc on 2 nm tetracene (Tc); ( b ) 2 nm CuPc on 20 nm Tc; ( c ) 15 nm CuPc only; and ( d ) 20 nm of Tc only. The colour scale represents photoemission intensity (normalized). All spectra were recorded with h ν 1 =2.43 eV and h ν 2 =4.65 eV. The inset in c shows TR-2PPE spectra for the 15-nm CuPc thin film excited at h ν 1 =1.96 eV and probed at h ν 2 =4.65 eV. Full size image To assign the CT peak, it is first necessary to identify components from isolated CuPc and Tc thin films. Figure 3c,d shows TR-2PPE spectra from neat CuPc (15 nm) and Tc (20 nm) for the same excitation energies (hν 1 =2.43 eV, hν 2 =4.65 eV) as those in Fig. 3a,b. For CuPc, there is little absorption at 2.43 eV and we see negligible photoelectron intensity. For comparison, when the CuPc layer is selectively excited at the absorption peak of hν 1 =1.96 eV, TR-2PPE spectrum reveals the short-lived S 1 centred at around −3.85 eV, which converts to T 1 in ~0.5 ps (inset in Fig. 3c ). For neat Tc (Fig. 3d), excitation at hν 1 =2.43 eV results in an S 1 -ME quantum superposition state, giving rise to photoemission intensities at the T 1 (−4.35 eV) and S 1 (−3.25 eV) positions [17] . The initial fast decay (≤1 ps) in both S 1 and triplet pair intensities for Tc excited at above threshold photon energies have been attributed to excitation localization dynamics, which decreases the ionization cross-section [17] . The transient peak from the bilayer spectra in Fig. 2a,b approximately between −3.8 and −3.3 eV (centred around −3.6 eV) is energetically located in between the S 1 state in CuPc (−3.85 eV) and that in Tc (−3.25 eV). The decay of this broad peak (2.6±0.5 ps) is much slower than the sub-ps dynamics of intersystem crossing in CuPc ( Fig. 2c , inset) or the initial 2PPE intensity decay dynamics in Tc ( Fig. 2d ) [17] . We can conclude that the transient CT peak in Fig. 3a,b cannot be due to overlapping intensities from Tc S 1 or from CuPc S 1 alone, but must substantially involve a contribution specific to the CuPc/Tc interface. We assign this mainly to a CT exciton resulting from the dissociation of the initially populated Tc S 1 exciton at its interface with CuPc. Note that the broad CT peak from the 2-nm/20-nm CuPc/Tc sample is slightly higher in relative intensity (~20%) and less resolved from the T 1 peak than that from the 2-nm/2-nm sample (see Supplementary Fig. S1 for vertical cuts at different time delays). We may attribute this difference to different contributions of overlapping spectral features from Tc S 1 and CuPc S 1 ; the latter is formed via Förster resonant energy transfer from the initially excited Tc S 1 exciton. Supporting the assignment of the CT state, we note that the rise in its populations is delayed, as shown in Fig. 4 for the 2-nm/20-nm CuPc/Tc sample (similar results are obtained for the 2-nm/2-nm CuPc/Tc sample, Supplementary Fig. S2 ). We integrated the photoemission intensities in the following spectral windows to improve signal-to-noise ratio and minimize spectral overlap: −2.7 to –3.0 eV for Tc S 1 and −3.5 to –3.8 eV for the CT state. The intensity of the Tc S1 state (red) rises with the laser pulse; the decay initially is on a sub-ps timescale and slows by more than one order of magnitude at longer times ( Supplementary Fig. S1 ) [17] . In contrast to that of Tc S 1 , there is a clear delay in the rise of CT peak intensities (blue curve); the CT state rises with a time constant of 400±100 fs attributed to electron transfer from photoexcited Tc to CuPc. It subsequently decays on the timescale of 2.6±0.5 ps. Details on kinetic analysis that yielded the time constants are presented below. Importantly, the decay in CT exciton intensity does not lead to the rise in the populations of other excitonic states (for example, CuPc T 1 states). We conclude that the decay of CT exciton population results from charge recombination, as expected from tightly bound interfacial CT excitons in the absence of competitive channels for further charge separation [21] . As the CT rate (400 fs) −1 is more than one order of magnitude faster than that of singlet fission (7 ps) −1 in Tc, the formation and decay of CT excitons at the Tc/CuPc interface represents a loss channel for solar energy conversion. Note that CT states for the two bilayer samples appear different in the pseudo-colour plots in Fig. 3a,b because of changes in the relative peak intensities ( Supplementary Fig. S2 ). 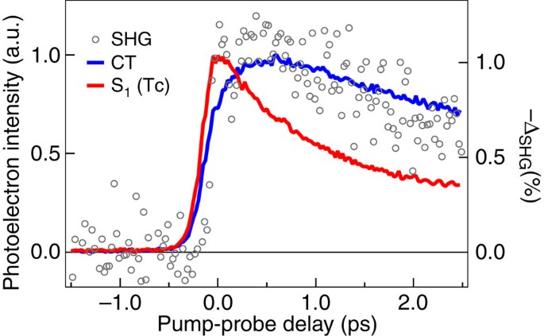Figure 4: Pump-probe time profiles of photoemission intensities and SHG signal. Integrated TR-2PPE intensities (left axis), −2.7 to −3.0 eV for Tc S1(red) and −3.5 to −3.8 eV for the CT state (blue) as a function of pump-probe delay time from the 2-nm/20-nm CuPc/Tc interfaces. Also shown is a TR-EFISH profile (grey circles, right axis) obtained for a 20-nm/20-nm CuPc/Tc interface. The pump photon energy is hν1=2.43 eV in TR-2PPE and hν1=2.41 eV in TR-EFISH. Figure 4: Pump-probe time profiles of photoemission intensities and SHG signal. Integrated TR-2PPE intensities (left axis), −2.7 to −3.0 eV for Tc S 1 (red) and −3.5 to −3.8 eV for the CT state (blue) as a function of pump-probe delay time from the 2-nm/20-nm CuPc/Tc interfaces. Also shown is a TR-EFISH profile (grey circles, right axis) obtained for a 20-nm/20-nm CuPc/Tc interface. The pump photon energy is hν 1 =2.43 eV in TR-2PPE and h ν 1 =2.41 eV in TR-EFISH. Full size image As an independent verification of the CT states, we turn to a complementary technique, time-resolved electric field-induced second harmonic generation (TR-EFISH). EFISH [22] , [23] is a four-wave mixing process: two optical fields at frequency ω mix with a direct current field to give signal at frequency 2 ω . We have successfully implemented this in the time-resolved mode to detect transient electric fields resulting from charge separation at donor/acceptor interfaces [21] , [24] , [25] , [26] , [27] . The open circles in Fig. 4 show TR-EFISH spectrum from a 20-nm/20-nm CuPc/Tc sample pumped at hν 1 =2.41 eV and probed at hν 2 =1.53 eV (second harmonic generation (SHG) at 3.06 eV). Pump-induced change in SHG intensity is clearly observed, with the rise and decay dynamics in excellent agreement with those of the CT peak intensity from TR-2PPE. In control experiments, we show the absence of pump-induced change in SHG intensity for CuPc or Tc only excited at hν=2.41 eV ( Supplementary Fig. S3 ). Thus, the pump-induced SHG response in Fig. 4 results specifically from the CuPc/Tc interface and is assigned to EFISH because of CT. The excited-state electron transfer to form the CT exciton state should be efficient, given the energetic alignment in Fig. 2d . The CT state is ~0.25 eV higher in energy than that of CuPc S 1 ; this is expected because a CT exciton should have a lower binding energy than that of the S 1 state because of an increased charge separation in the former. Note that the CT exciton is energetically broad, and this may be attributed to a distribution of CT exciton-binding energies due to different e–h distances and molecular orientations at the interface. Given the presence of this CT exciton formation and recombination channel, we predict that, for the efficient transfer of triplet excitons resulting from singlet fission, the excitation must be initiated away from the A/B interface so that singlet fission can become more competitive than singlet diffusion to the A/B interface and dissociate to the CT excitons. This is indeed observed for a thicker Tc underlayer, as detailed below. Triplet energy transfer Although the bilayer samples with different Tc thicknesses (2 versus 20 nm) show similar dynamics on short times ( Fig. 3 , ), they are distinctively different on longer timescales. 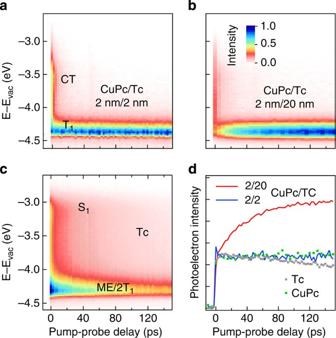Figure 5: Pseudo-colour plots of TR-2PPE spectra in 150 ps. (a) A 2nm CuPc on 2 nm Tc; and (b) 2 nm CuPc on 20 nm Tc. The colour scale is photoemission intensity (normalized). (c) TR-2PPE spectra from a 20nm Tc thin film. All spectra were recorded with hν1=2.43 eV and hν2=4.65 eV. (d) Photoemission intensities of the triplet states as a function of pump-probe delay times: 2 nm/2 nm (blue curve) and 2 nm/20 nm (red curve) CuPc/Tc interfaces; 20 nm Tc only (grey dots); 15 nm CuPc only excited at hν1=1.96 eV (green dots). Figure 5a,b shows pseudo-colour plots of TR-2PPE spectra for the two bilayer samples up to a pump-probe delay of 160 ps. The T 1 population is nearly constant for the CuPc/Tc sample with 2 nm Tc, whereas that from 20 nm Tc interface shows a large T 1 population increase over this time window. For comparison, Fig. 5c shows TR-2PPE spectrum for Tc only, without the CuPc overlayer. For Tc, there is an equilibrium between singlet and triplet pair states owing to the quantum superposition on short timescales (7 ps) and to triplet–triplet annihilation on longer times; the triplet population decays on this timescale mainly because of radiative recombination (fluorescence emission) [15] , [16] , [17] . Figure 5d summarizes the triplet populations as a function of pump-probe delays for the 2-nm/20-nm CuPc/Tc sample (red line), 2-nm/2-nm CuPc/Tc (blue line) and 20-nm Tc only (grey dots), all exited at hν 1 =2.43 eV. For comparison, we also include neat CuPc directly excited with photon energy of hν 1 =1.96 eV. Note that the triplet peak intensity is a sum of contributions from both Tc and CuPc near the interface for bilayer samples because the two states are nearly resonant. Although the neat Tc sample shows a slow decay in triplet population with time, both neat CuPc and the bilayer sample with a 2-nm Tc underlayer show constant triplet population on this timescale. The CuPc triplet is much longer lived than that of Tc. The constant T 1 population from the 2-nm CuPc/2-nm Tc sample suggests that triplets from the population of S 1 in Tc that has escaped the charge separation/recombination loss channel are successfully transferred to CuPc. In contrast to the other three samples, the 2-nm/20-nm CuPc/Tc sample shows a slow rise in triplet population. In this case, singlet fission is competitive only for excitations in Tc away from the CuPc/Tc interface and the resulting triplets are transferred to CuPc through Dexter energy transfer [28] , that is, direct intermolecular electronic coupling. Figure 5: Pseudo-colour plots of TR-2PPE spectra in 150 ps. ( a ) A 2nm CuPc on 2 nm Tc; and ( b ) 2 nm CuPc on 20 nm Tc. The colour scale is photoemission intensity (normalized). ( c ) TR-2PPE spectra from a 20nm Tc thin film. All spectra were recorded with hν 1 =2.43 eV and hν 2 =4.65 eV. ( d ) Photoemission intensities of the triplet states as a function of pump-probe delay times: 2 nm/2 nm (blue curve) and 2 nm/20 nm (red curve) CuPc/Tc interfaces; 20 nm Tc only (grey dots); 15 nm CuPc only excited at hν 1 =1.96 eV (green dots). Full size image We now carry out kinetic analysis to determine the relative rates of charge and energy transfer at the CuPc/Tc interface. We consider the initially populated S 1 ME coherent superposition [17] as a single entity, [SM]. The competitive time constants of singlet fission, τ SF , and of CT, τ CT , draw from this shared population. Singlet fission leads to population of the Tc T 1 , which acts as a reservoir for energy transfer to CuPc T′ 1 , with time constant τ TET . CT results in population of the CT state, which decays with time constant τ RC . Writing out the populations we have, where I hυ1 ( t ) is the excitation laser pulse multiplied by the excitation cross section (assumed to be of Gaussian shape) that initially populate the Tc S 1 ME superposition state. The time constant of singlet fission is fixed at τ SF =7ps, as determined in our TR-2PPE experiments [11] , [17] . We fit the parameters τ CT and τ RC to the rise and decay of the CT state in both bilayer samples, and τ TET to the slow rise in CuPc T′ 1 population from the 2-nm CuPc/20-nm Tc sample, as shown in Fig. 6 . Note that in both sets of data, background signals attributable to photoemission from the underlying Tc have been subtracted. The fits yield time constants of τ CT =400±100 fs, τ RC =2.6±0.5 ps and τ TET =45±5 ps. The electron transfer time constant of 400±100 fs from the Tc S 1 to CuPc is nearly identical to those of electron transfer from photoexcited pentacene [27] or Tc (ref. 17 ) to C 60 , suggesting similar electronic coupling constants at these van der Waals interfaces. The singlet fission process in Tc (7 ps) [11] , [17] is more than one order of magnitude slower than that of electron transfer at the interface and is not competitive with the charge separation and recombination channel. Thus, only Tc S 1 located away from the interface can undergo fission, followed by triplet diffusion (Dexter energy transfer) to CuPc on a 45±5-ps timescale. Note that the above kinetic analysis should be treated as a semiquantitative estimation. A more accurate treatment would require the inclusion of back reactions to re-form the singlet from the triplet pair in Tc, direct singlet energy transfer from Tc to CuPc and intersystem crossing in CuPc. 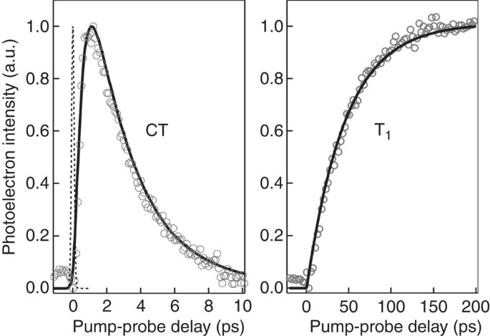Figure 6: Kinetics of CT formation/decay and triplet energy transfer. Photoemission intensity of the interfacial CT exciton (left) and CuPc T′1exciton (right) as a function of pump-probe delay for 2 nm CuPc on 20 nm Tc. The circles are experimental data points and the solid lines are fits to the kinetic model in equations (1)–(4),. The dashed curve in the right panel is the instrument response function (2PPE pump-probe cross correlation obtained from an occupied state of Au). Figure 6: Kinetics of CT formation/decay and triplet energy transfer. Photoemission intensity of the interfacial CT exciton (left) and CuPc T′ 1 exciton (right) as a function of pump-probe delay for 2 nm CuPc on 20 nm Tc. The circles are experimental data points and the solid lines are fits to the kinetic model in equations (1)–(4),. The dashed curve in the right panel is the instrument response function (2PPE pump-probe cross correlation obtained from an occupied state of Au). Full size image The intensity of the T 1 peak is approximately one order of magnitude higher than that of the CT peak. Although we cannot quantitatively convert these intensities to populations because of the absence of knowledge on photoionization cross-sections (that is, the second step in TR-2PPE), the results suggest qualitatively that more S 1 states away from the interface in the 20-nm Tc thin film undergo singlet fission and subsequent triplet transfer to CuPc than those lost because of charge separation and recombination. Given the singlet exciton diffusion length of 12 nm (in the direction perpendicular to the a–b plane in Tc) [29] and the light attenuation length in Tc of λ a ~100 nm at hν 1 =2.43 eV (ref. 15 ), we estimate that 24% of the singlet excitons within the 20-nm film can diffuse to the interface with CuPc for charge separation and recombination, whereas 76% can undergo singlet fission. The percentage of the CT loss channel increases as the thickness of the singlet fission layer decreases. This argues against the use of the most popular bulk heterojunction architecture [30] for the implementation of singlet in organic photovoltaics. In principle, one can increase the thickness of the singlet fission layer in the trilayer structures ( Fig. 1 ) to minimize the CT/recombination loss channel at the donor/donor interface ( Supplementary Fig. S4 and equation (5)). However, a thick singlet fission layer introduces additional challenges, such as limited hole mobility or charge trapping and competing long range Förster resonance energy transfer directly from the singlet state. We show, using the CuPc/Tc bilayer model system and TR-2PPE spectroscopy, the critical competition between (1) singlet fission/triplet energy transfer and (2) singlet dissociation/charge recombination at the interface. For Tc, where singlet fission occurs on a timescale of 7 ps, electron transfer at the CuPc interface is more competitive with CT exciton formation in 400±100 fs and recombination in 2.6±0.5 ps. The presence of this charge separation and recombination process is a power loss channel, which is unfortunately a result of the energetic requirement for efficient triplet energy transfer. The T 1 state of the singlet fission material absorbing at the blue end of the solar spectrum must be slightly higher in energy than that of the second chromophore absorbing at the red end. As a result, the S 1 state in this second chromophore must be significantly lower in energy than that of the singlet fission material (see Fig. 1 ). This arrangement makes interfacial CT state formation favourable. To minimize the CT channel, one must reduce the interfacial area between the two chromophores, for example, by using bilayer structures with a relatively thick singlet fission layer. The thickness of this layer must also be judiciously chosen to balance light absorption, triplet diffusion and transfer at the interface, triplet–triplet annihilation and competing singlet energy transfer. These competing dynamic channels put stringent requirements on the design of materials and interfaces for the most efficient harvesting of triplet excitons from singlet fission in solar energy conversion. Sample preparation for TR-2PPE experiments All organic thin film samples were prepared in situ in an ultra high vacuum chamber (base pressure 10 −9 Torr), with film thickness calibrated with a quartz crystal microbalance. We started with a single crystal Au(111) surface (1 cm diameter) prepared using standard argon ion sputtering and annealing (three cycles: Ar + 10 μA cm −2 for 20 min, 773 K for 60 min). A five monolayer epitaxial C 60 film (Sigma-Aldrich, 99.9% purity) was deposited onto the Au(111) surface from Knudsen cell to produce a (2 × 2 ) R30° super lattice, as confirmed by low-energy electron diffraction [31] . Tc (Sigma-Aldrich, 99.99% purity) was vapour deposited from a Knudsen cell onto the fullerene-covered Au(111) surface at a sample temperature of 298 K and a growth rate of 1 Å s −1 . The presence of fullerene reduces interaction between Tc and the surface and results in a bulk-like Tc thin film, as described by Dougherty et al . [32] for pentacene on fullerene-covered Au(111). A subsequent layer of CuPc (Sigma-Aldrich 99.9%) was vapour deposited from a Knudsen cell onto the Tc surface at 298 K and a deposition rate of 1 Å s −1 . Each sample was transferred in situ to a separate ultra high vacuum analysis chamber with a base pressure of 1 × 10 −10 Torr. Characterization of the samples by atomic force microscopy ( ex situ ) showed small clusters (a few nm to ~10 nm sizes) of CuPc on top of flat terraces (~500 nm) of Tc ( Supplementary Figs S5 and S6 ). TR-2PPE measurement The sample (at room temperature) was excited by a pump laser pulse (hν 1 =2.43 or 1.96 eV, pulse energy=2 nJ and width=100 fs) from the output of an optical parametric oscillator (Coherent Mira-OPO). The excited state was ionized by a time-delayed probe laser pulse (hν 2 =4.65 eV, pulse energy=0.25 nJ and pulse duration=140 fs), which was frequency tripled from the output of the Ti:sapphire oscillator (Coherent Mira-HP). A pair of Pockels cells (Conoptics 350-160-02) was utilized to decrease the repetition rate from 76 to 3.8 MHz and reduce the buildup of long-lived triplet excitons and/or trapped charges between laser pulses. The pump and probe laser beams were slightly focused and non-collinearly recombined on the sample surface at 45° with respect to the surface normal, to an elliptic spot of ~0.35 × 0.50 mm 2 . In ultraviolet photoelectron spectroscopy measurement, a helium discharge lamp (vacuum generator, He-I, hν=21.2 eV) was used in place of the laser pulses for photoionization. Photoelectrons were detected with a hemispherical electron analyser (VG-Scienta R3000). A small bias of −2.5 to 3.0 V was applied to the electrically isolated sample to aid in collection of the low-energy electrons. In all data presented here, the average pump laser power used was 7.6 mW. We carried out control experiments on the laser power dependence (2–20 mW) and verified that the photoemission intensities of all the excitonic states increased linearly with laser power, whereas the kinetic profiles were completely independent of pump laser power ( Supplementary Fig. S7 ). As detailed before in our previous publications, there was weak 2PPE signal (≤10%) in the triplet region before the arrival of the pump laser pulse [17] . The photoemission signal came from probe pulse only and could be attributed to trapped triplets between laser pulses. This background was subtracted from pump-probe spectra presented here. TR-EFISH experiments All organic thin films (20 nm Tc, 20 nm CuPc and 20 nm CuPc on 20 nm Tc) were thermally evaporated onto single crystal sapphire (0001) surfaces (MTI Corporation) in a vacuum chamber (10 −7 Torr). The deposition rates of Tc and CuPc were 0.02~0.03 and 0.01 nm s −1 , respectively, as monitored with a quartz crystal microbalance. The experimental set-up has been described in detail before [21] . Briefly, the laser pulses were from a femtosecond regenerative amplifier (Coherent REGA, 250 KHz, λ =810 nm) seeded by a homebuilt femtosecond Ti-Sapphire oscillator (810 nm, bandwidth 40 nm). The REGA output was split into two beams: one as the probe beam and the other as the pump of a tunable optical parametric amplifier (Coherent Vis-OPA, 500–750 nm). The 515-nm pump pulse (hv=2.41 eV, pulse energy=24 nJ) from the OPA and the 810-nm probe pulse (hv=1.53 eV, pulse energy=80 nJ) from the REGA were focused onto the sample surface with incident angles of 42° and 45°, respectively, with respect to the surface normal. The spot size was 0.01 mm 2 for the pump and 0.003 mm 2 for the probe. A half-wave plate was placed in the probe beam path to control the polarization, and the pump beam was fixed at the p -polarization. We optimized the temporal and spatial overlap of the pump and the probe pulses through measuring sum-frequency generation from each sample and the pulse widths were ~70 fs. The reflected SHG signal was collected by a photomultiplier tube after passing through a polarizer, a combination of filters and a monochromator. All TR-EFISH measurements were carried out in a N 2 -filled cryostat at room temperature. Note that, on each organic thin film sample, there was static SHG signal from the surface or interface in the absence of pump laser. The pump-induced change can increase or decrease the total SHG intensity depending on the phase relationship between the transient EFISH and static SHG components. In the case of the 20-nm/20-nm CuPc/Tc sample, the pump-induced transient EFISH component decreases the overall SHG intensity. The scale in Fig. 4 (right axis) is the percentage of pump-induced change in SHG intensity. Estimation of the CT loss channel Consider a trilayer solar cell structure illustrated in Fig. 1 with normal light incidence. The singlet fission Tc layer is on top, the CuPc layer is in the middle and the electron acceptor at the bottom. On the basis of the published absorption spectra of Tc thin films [15] , we calculate a light attenuation length in Tc of λ a =100 nm at hν 1 =2.43 eV. The singlet exciton diffusion length in the direction perpendicular to the herringbone a–b plane of crystalline Tc is λ d =12 nm (ref. 29 ). The thickness of the Tc layer is L . We assume that a singlet exciton diffuse in both directions perpendicular to the ab plane and that diffusion away from the interface to CuPc will not be considered for the CT channel (that is, no reflection). The percentage of singlet exciton, which diffuse to the interface with CuPc and undergo CT/recombination, is given by: Supplementary Fig. S4 shows the calculated results from equation (5) based on parameters for Tc. For a 20-nm thick Tc film, we obtain a value of 24% loss of singlet states in Tc to the charge separation/recombination channel. This loss increases to 50% as the Tc thin film thickness decreases. It decreases to 4% for a 100-nm thick Tc film. How to cite this article: Tritsch, J. R. et al . Harvesting singlet fission for solar energy conversion via triplet energy transfer. Nat. Commun. 4:2679 doi: 10.1038/ncomms3679 (2013).